Environmental conditions and community evenness determine the outcome of biological invasion Biological invasion is widely studied, however, conclusions on the outcome of this process mainly originate from observations in systems that leave a large number of experimental variables uncontrolled. Here using a fully controlled system consisting of assembled bacterial communities, we evaluate the degree of invasion and the effect on the community functionality in relation to the initial community evenness under specific environmental stressors. We show that evenness influences the level of invasion and that the introduced species can promote functionality under stress. The evenness–invasibility relationship is negative in the absence and neutral in the presence of stress. Under these conditions, the introduced species is able to maintain the functionality of uneven communities. These results indicate that communities, initially having the same genetic background, in the presence of the same invader, react in a different way with respect to invasibility and functionality depending on specific environmental conditions and community evenness. Biodiversity has been shown to significantly influence invasion in disparate aquatic and terrestrial environments [1] , [2] . Biodiversity correlates positively [3] , negatively [4] or neutrally [5] with the capacity of species to invade resident communities. Many factors, such as nutrient availability [3] , scale [6] , functional niches [7] , environmental stressors [8] , facilitation or competition [9] and biodiversity [10] can co-occur, driving the invasion process and influencing the final outcome. The available studies, mainly based on observations, do not take into account intrinsic system effects and a large number of non-controlled variables are present (climatic conditions, soil type, soil microbial community, presence of symbiotic or antagonistic partners and so on.) [11] , [12] . These confounding factors and the reciprocal interactions may lead to opposite conclusions on the role of a specific parameter, even in closely related ecosystems [4] , [5] . Experiments conducted under controlled conditions give the opportunity to target some of these confounding factors, eventually explaining the inter-system variability, despite the fact that this approach is a simplification of the reality. In this study, we applied the approach used by Wittebolle et al ., [13] which is well suited for validating ecological theories and can be run under fully controlled conditions. The effect of an introduced species (termed the ‘invader’) on ecosystem functionality was investigated in relation to the initial evenness of the native community. We decided to focus on evenness and to maintain a high level of richness because natural and anthropogenic activities primarily influence the relative abundance of species long before a species is threatened by extinction [14] , [15] . Rationale of the experimental setup The impact of initial community evenness on invasibility and the effect of the invader on the functionality of the resident community, that is, denitrification, were assessed by the use of assembled denitrifying bacterial communities. To exclude other confounding factors that could influence invasion, our tests were conducted with a complex medium to avoid nutrient limitation, an assembled community composed of bacteria occupying the same functional niche (the capability for nitrite respiration), isolated from the same sample of homogenized activated sludge and without prior history of adaptation to prevailing environmental conditions, and an invader incapable of denitrification. A total of 17 denitrifying strains from four phyla ( Supplementary Table S1 ) were mixed in different proportions to create 3,192 microcosms ( Supplementary Data 1,2 ) with different levels of initial evenness but with the same richness. This number of strains represents a high richness, which ensures a good functionality [15] ; the complete range of evenness, expressed by the Gini coefficient (that is, 0 being a complete even community and 1 the most uneven community), was covered ( Supplementary Fig. S1 ). The microcosms were arranged in 96-well plates and incubated under two distinct conditions: no stress and salinity stress. Salinity stress was chosen, because it cannot be readily altered by the microorganisms and was shown to have a significant impact on the functionality of the community [16] . An open ecosystem (that is, a system that has an input of matter, for example, microorganisms [17] ) was simulated by challenging the assembled community with an introduced gfp -tagged, salt-resistant, non-denitrifying species—the invader—at a concentration of 0.1 and 1% of the initial total cell number ( Supplementary Fig. S2 ). In contrast, the control experiment with no introduced species simulated a closed ecosystem. After 20 h of anaerobic incubation, the percentage of nitrite removal was used as a measure of functionality of the community. The total number of cells and the number of gfp -tagged invader cells were analysed by flow cytometry to determine the invasion coefficient and the resident community cell number. The invasion coefficient, ranging from 0 (not invaded) to 1, corresponds to the proportion of invader cells to the total cell count, while the community cell count (CC community ) is equal to the total number of cells subtracted by the number of invader cells. Each of the response variables—functionality, invasion and CC community —has been analysed with additive quantile regression models [18] . By design, all of the models included terms for the row, column and plate effects. 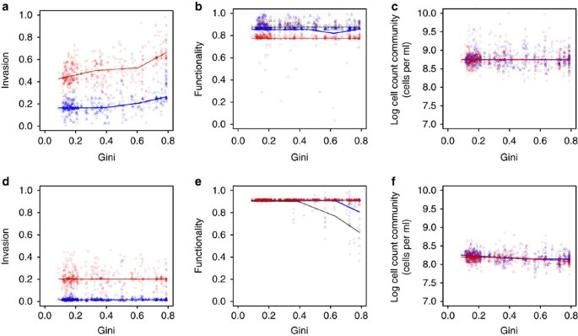Figure 1: Invasion in the absence and presence of salinity stress. The individual plots show invasion (a,d), its effect on functionality (b,e) and the growth of the community (c,f) in relation to the Gini coefficient in the absence (a–c) and presence (d–f) of salinity stress. Black crosses, blue triangles and red squares indicate the residuals at an initial invader concentration of 0, 0.1 and 1%, respectively, after correction for the row, column and plate effects. Black (0%), blue (0.1%) and red (1%) lines show the fits after model selection (Table 1). The effect of the Gini coefficient was modelled non-parametrically with a smoother spline, either unconstrained or with a monotonicity constraint (increasing or decreasing) ( Table 1 ). Table 1 Model selection for the three response variables. Full size table Invasion in the absence of stress Under different environmental conditions, the intrinsic characteristics of a microbial community influence its susceptibility to invasion and its functional stability. In the absence of salt, invasion increased with an increasing Gini coefficient ( Fig. 1a ) and was observed both at a low and high initial concentration of the invader: 0.1% ( P <0.001) and 1% ( P <0.001) of the total cell count, respectively, ( Supplementary Table S2 ). A higher initial concentration of the introduced strain produced a higher level of invasion ( P <0.001). The presence of the invader affected the performance of the community by lowering the overall denitrifying functionality ( P <0.001), independent of the degree of evenness ( Fig. 1b ) without influencing the growth of the community ( Fig. 1c ). Therefore, under conditions of no stress, the Gini coefficient was positively correlated with the degree of invasion and neutrally correlated with the CC community . Figure 1: Invasion in the absence and presence of salinity stress. The individual plots show invasion ( a , d ), its effect on functionality ( b , e ) and the growth of the community ( c , f ) in relation to the Gini coefficient in the absence ( a – c ) and presence ( d – f ) of salinity stress. Black crosses, blue triangles and red squares indicate the residuals at an initial invader concentration of 0, 0.1 and 1%, respectively, after correction for the row, column and plate effects. Black (0%), blue (0.1%) and red (1%) lines show the fits after model selection ( Table 1 ). Full size image Invasion in the presence of stress In the presence of salt ( Fig. 1d ), the degree of evenness did not influence the invasibility of the community ( P =0.86 and P =0.99 for 0.1% and 1% invader, respectively). However, the functionality of the community was strongly influenced by the introduction of the invader ( P <0.001) ( Fig. 1e ). Under salinity stress and in the absence of invasion, nitrite was only partially reduced by the denitrifying communities with a high Gini coefficient. These data confirmed what was previously shown, that communities with a high initial evenness have a higher potential to counteract the effect of a sudden selective stress than communities with a low initial evenness [16] . If the same communities were exposed to an invader, no negative correlation between functionality and the Gini coefficient was observed. The functionality was maintained at a high level over the complete range of evenness if the communities were challenged with the highest invader concentration. Similar to the effect observed under the conditions without salt, the presence of the invader under the stress condition had no effect on community growth ( P =0.365) ( Fig. 1f ). The functionality of invaded communities was always lower under non-stressed conditions compared with stress conditions ( P <0.001), while invasion was higher under non-stressed conditions and community growth was similar, all independently of the degree of evenness ( Supplementary Fig. S3 ). Several previous studies attempted to correlate invasion with the composition of the invaded community and some of these studies experimentally addressed the effect of invasion on ecosystem functioning [19] . In our work, the degree of evenness was negatively correlated with the susceptibility of the community to invasion in the absence of an external stress, as previously shown in grassland communities [4] , [20] , [21] . However, under stress conditions, the evenness–invasibility relationship became neutral, and the invasion potential was only associated with the initial amount of the invader. The effect of invasion on the functionality depended strongly on the environmental conditions: the functionality at a high Gini coefficient was enhanced under stress and lowered under non-stress conditions. The diversity–invasibility hypothesis states that a high species richness confers a high degree of invasion resistance [22] . However, it has also been reported that a positive relationship between diversity and invasibility can occur [3] , [6] , [10] . In the present study, we found that, even at a fixed high richness, the relative abundance of the species (that is, evenness) is an essential factor that determines the invasibility of the community ( Fig. 1a ). This effect can be explained by the potential niche overlap for carbon sources between the community and the invader. As shown in Fig. 2 , the niche overlap (consumption of carbon sources) was much higher with an even community as compared with most of the uneven mixes. Therefore, invasion is facilitated in uneven communities. In addition to biodiversity, environmental stress influenced the invasion potential. In fact, the level of invasion in two identical communities (same richness, evenness and species composition) in the presence of the same resources depended strictly on the presence of a stress. 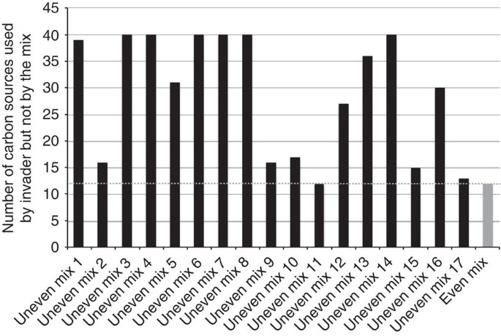Figure 2: Niche overlap of the available carbon sources. Number of carbon sources available for the invader that are not used by the even (grey bar)/uneven (black bars) mixes. The grey dotted line represents the level of carbon consumption of the even mix. The amount of available carbon sources for the invader—which was able to use 40 out of 95 carbon sources—was much lower with an even community as compared to most of the uneven mixes. Figure 2: Niche overlap of the available carbon sources. Number of carbon sources available for the invader that are not used by the even (grey bar)/uneven (black bars) mixes. The grey dotted line represents the level of carbon consumption of the even mix. The amount of available carbon sources for the invader—which was able to use 40 out of 95 carbon sources—was much lower with an even community as compared to most of the uneven mixes. Full size image Current debate also focuses on the effect of the invasion of an ecosystem on the functioning of the system [23] , [24] , [25] . In this study, we confirmed that the degree of evenness is a key element for preserving the overall functionality in a closed community [16] . In fact, the functionality of an even community could be maintained under both stressed and non-stressed conditions. Conversely, the functional stability of a highly uneven community is endangered by salinity stress ( Fig. 1e , black line). The same effect on functionality was also observed in an open community. In this situation, however, the overall functionality of an uneven community was preserved at high levels of the invader, although the introduced species, a non-denitrifier, made no direct contribution to the existing functionality ( Fig. 1e , red line). This result suggests that a closed system is sensitive to functionality loss when exposed to fluctuating environmental conditions [13] , [26] ( Fig. 3 , bottom right). An open system in which non-native species have the ability to invade the resident community may be more resistant to stress than a closed system and can maintain or even improve its functionality when an invader is present. 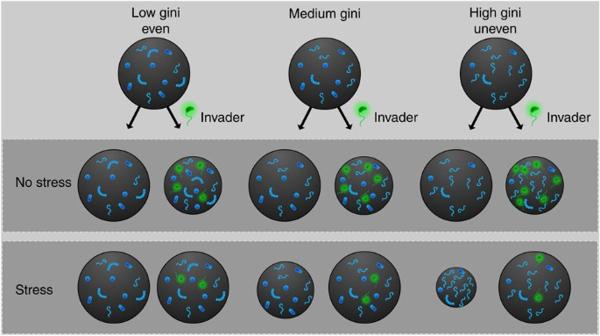Figure 3: Graphical summary of the main observations. Microcosms, composed of seventeen denitrifying strains (blue cells, different shapes), have been assembled with different levels of initial evenness (different proportion of cells), from a low to high Gini coefficient. These microcosms were challenged with a non-denitrifying invader (green cells) under stressed and non-stressed conditions. The ecosystem functionality (size of circles) and invasibility (number of green cells) were measured. Invasion was generally lower in the presence of salt stress than in the absence of salt. Under no-stress conditions, the presence of the invader negatively affected the community and its functionality, whereas the same relationship was positive under stress conditions. Figure 3: Graphical summary of the main observations. Microcosms, composed of seventeen denitrifying strains (blue cells, different shapes), have been assembled with different levels of initial evenness (different proportion of cells), from a low to high Gini coefficient. These microcosms were challenged with a non-denitrifying invader (green cells) under stressed and non-stressed conditions. The ecosystem functionality (size of circles) and invasibility (number of green cells) were measured. Invasion was generally lower in the presence of salt stress than in the absence of salt. Under no-stress conditions, the presence of the invader negatively affected the community and its functionality, whereas the same relationship was positive under stress conditions. Full size image Our aim was to evaluate what could be the impact of human activities—that tend to modify the composition of natural communities—on invasibility and functionality under different environmental conditions. We showed that the same community, with the same genetic background, in the presence of the same invader behaved differently depending on specific environmental conditions and its evenness. Despite our conclusions rising from these observations are firstly pertinent to our ecological system, we suggest to consider it as a possible interpretation model that could have analogies in other systems including the macro-ecology systems. Under stress conditions an invasive species can preserve the indigenous functionality, whereas under non-stress conditions the functionality can be threatened. In the latter case evenness has a crucial role in determining the community resistance to invasibility and in preserving ecosystem functionality. Thus, on the one hand, invasion can support ecosystem resilience and services [24] , whereas on the other hand, it can be considered negative towards conservation biology [23] , [25] . Hence, in case of putative imposition of ecological management, both potential impacts of invasion warrant careful consideration. Experimental design In this study, we used 210 mixtures with different evenness values, corresponding to unique Gini and dominant species combinations. These mixtures were created following a stochastic exchange search algorithm for D -optimal designs [27] according to the following procedure. The first step was the random construction of a design. The relative abundances of the 17 species were randomly assigned. Five 96-well plates were randomly filled with the mixtures, with adjacent duplicates of each mixture. Negative controls were positioned in the centre and the corners of each plate to assess potential row, column and plate effects. We computed the D -optimality criterion for this random design and a linear model, with factor effects for the row, column, invader and salt stress, a random effect for the plate, and a linear and quadratic effect of for the Gini. In the next step, the mixtures were randomly exchanged between positions and plates, and the D -optimality criterion was computed for each new design; this procedure was repeated 1,000 times. The best design with the largest D -optimality criterion was selected as the quasi D -optimal design. The complete procedure, starting from the construction of the random design, was also repeated 10,000 times. From the 10,000,000 evaluated designs, the design with the largest D -optimality criterion was selected for this study. During the optimization process, the convergence of the D -optimality criterion was monitored to ensure that the final selected design was sufficiently well converged. Laboratory methods A chromosomally gfp -tagged Pseudomonas sp. and 17 denitrifying strains ( Supplementary Table S1 ) were stored in ready-to-use aliquots at −80 °C. For each experiment, the strains were cultured for 48 h and subcultured for 40 h in trypticase soy broth at 28 °C under aerobic conditions to obtain actively growing microorganisms. The denitrifying strains were diluted to 10 7 cells ml −1 and the invader to 1.5 × 10 7 cells ml −1 , as measured by flow cytometry (CyAn ADP LX, Dako, Heverlee, Belgium). Communities with different degrees of initial evenness were created by mixing the diluted denitrifying strains in different proportions. Each mixture was divided into three aliquots. No cells of the invader were added to the first aliquot (0% invader); to the second and third aliquot, the invader was added so that the number of invader cells in the mixtures was 0.1 and 1% of the total number of cells, respectively. These mixtures were used to assemble microcosms in duplicate in multiwell plates, according to the design, using a BioRobot 3000 (Qiagen, Venlo, The Netherlands). The mixtures were 1:1 diluted in trypticase soy broth supplemented with 12 mM nitrite and optionally supplemented with 4% (w/v) NaCl (for the salinity stress) to obtain a final concentration of 6 mM nitrite and 2% NaCl. The plates were incubated anoxically for 20 h at 28 °C, and the optical density (620 nm) was measured. The relative abundance of the invader cells and the total cell count of the invaded communities were determined by flow cytometry, and the residual nitrite concentration was determined with the Montgomery reaction. In order to identify a potential niche overlap, an anaerobic metabolic fingerprint (using 95 different carbon sources of the Biolog AN microplate (Hayward, USA) and 6 mM nitrite as electron acceptor) was made for 17 uneven communities (each with one different dominant strain), the perfectly even community and the invader. For each mix, we determined the unique available carbon sources for the invader by subtracting the carbon sources used by a single mix from those used by the invader itself. Statistical analysis Each of the response variables (functionality, invasion and CC community ) has been analysed with additive quantile regression models [18] . A separate analysis was performed for each invader/salt combination. The Gini effect was modelled non-parametrically using a smoother spline, either unconstrained or with a monotonicity constraint (increasing or decreasing). The smoothing parameter was optimized by minimizing the Akaike’s Information Criterion. All hypothesis tests were based on generalized likelihood ratio tests performed at the 5% level of significance. For forward model selection the testing sequence was: (1) no Gini effect versus a monotonic Gini effect (increasing or decreasing, depending on the Akaike’s Information Criterion), (2) monotonic Gini effect versus an unconstrained Gini effect. Additive quantile regression models have been used to analyse the response variables at the 50, 10 and 90% quantiles. Quantile regression extends ordinary regression models in the sense that a particular quantile of the conditional response distribution is modelled instead of the mean [28] . The choice for this method is motivated by the variable shapes of the conditional response distributions as a function of the Gini coefficient. Results of the Gini effects are only reported for the analyses at the 50% quantile (median), unless Gini effects were only established at the 10% or 90% quantiles. Analyses were conducted with the quantile set at either 50% (invasion and CC community ) or 10% (functionality). The partial residuals, shown in the graphs of the model fits, were always constructed relative to the 50% quantile regression model that corrects for row, column and plate effects. The axis of the residuals of the functionality and invasion response variables were rescaled to obtain values between 0 and 1, with 0 the lowest and 1 the highest measured value. How to cite this article: De Roy, K. et al . Environmental conditions and community evenness determine the outcome of biological invasion. Nat. Commun. 4:1383 doi: 10.1038/ncomms2392 (2013).